RETRACTED ARTICLE: Sulfur availability regulates plant growth via glucose-TOR signaling 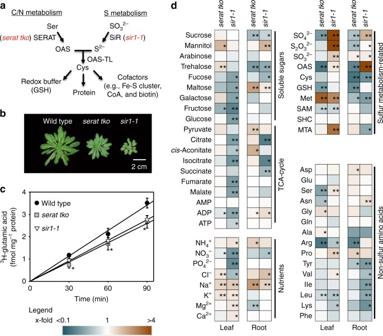Fig. 1 Limitation of OAS or sulfide for Cys biosynthesis results in decreased translation and distinct metabolic phenotype.aMetabolic pathway of cysteine biosynthesis.bRosette phenotype of 7-week-old wild-typeserat tkoandsir1-1grown in hydroponic culture. Scale bar, 2 cm.cGlobal translation rate in different genotypes as determined by time-resolved incorporation of3H-glutamic acid into proteins (n= 3, mean ± s.e.m., one-way ANOVA, *p< 0.05).dRelative fold change of metabolites is depicted as a heat map in cysteine-synthesis-depleted mutants compared to wild type (n= 3–4, one-way ANOVA, *p< 0.05, **p< 0.01) Growth of eukaryotic cells is regulated by the target of rapamycin (TOR). The strongest activator of TOR in metazoa is amino acid availability. The established transducers of amino acid sensing to TOR in metazoa are absent in plants. Hence, a fundamental question is how amino acid sensing is achieved in photo-autotrophic organisms. Here we demonstrate that the plant Arabidopsis does not sense the sulfur-containing amino acid cysteine itself, but its biosynthetic precursors. We identify the kinase GCN2 as a sensor of the carbon/nitrogen precursor availability, whereas limitation of the sulfur precursor is transduced to TOR by downregulation of glucose metabolism. The downregulated TOR activity caused decreased translation, lowered meristematic activity, and elevated autophagy. Our results uncover a plant-specific adaptation of TOR function. In concert with GCN2, TOR allows photo-autotrophic eukaryotes to coordinate the fluxes of carbon, nitrogen, and sulfur for efficient cysteine biosynthesis under varying external nutrient supply. Plants continuously decide how to balance the use of their acquired resources for growth or for stress responses, since they must compete with their neighbors for acquisition of nutrients by developmental plasticity and they must fight environmental challenges on site. Protein turnover causes up to 50% of total energy costs in fast growing cells [1] . Consequently, one immediate reaction of cells to various stresses, including nutrient starvation, is translation arrest. This thereby releases energy and resources for stress responses. Besides numerous regulatory events for selective translation and direct modification of the ribosome subunits that affect mRNA binding via the Cap-binding proteins, translation is regulated in eukaryotes frequently via two processes: formation of the translational pre-initiation complex and rRNA transcription for ribosome biogenesis reviewed in refs. [2] , [3] , [4] . Formation of the pre-initiation complex is mainly triggered by phosphorylation of the eukaryotic initiation factor 2α (eIF2α). eIF2α is phosphorylated in mammals by four sensor kinases (GCN2, PERK, PKR, and HRI), which are activated by diverse stresses defining eIF2α phosphorylation as a hotspot of stress-induced translation control. Out of the four mammalian eIF2a kinases, only GCN2 (general control non-derepressible 2) is conserved in plants [5] , [6] . It is selectively stimulated by amino acid depletion in plants, fungi, and metazoan and is mandatory for pathogen-induced growth arrest via beta-aminobutyric acid [7] , [8] , [9] . The biogenesis of ribosomes is regulated in all eukaryotes by the highly conserved sensor–kinase TOR (target of rapamycin) [3] , [10] . In addition to ribosome biogenesis, TOR controls cell-cycle progression, cell growth and autophagy in animals, yeast and plants, making TOR the master regulator of growth in autotrophic and heterotrophic eukaryotes [3] , [11] , [12] . In plants, TOR is known to balance growth with carbon availability by affecting brassinosteroid signaling [13] and to control life span [14] . It furthermore regulates translation re-initiation of uORF-containing mRNAs [15] and triggers stress responses by phosphorylation of its downstream target S6 kinase [16] . Xiong et al. coined the term glucose-TOR (Glc-TOR) signaling to describe control of TOR activity by glucose through glycolysis and mitochondrial bioenergetics to regulate meristem activation. Recent reviews describe the role of plant TOR in autophagy regulation, auxin sensing, development, and nutrient sensing [17] , [18] , [19] , [20] . In animals, TOR perceives systemic signals like growth factors and local signals like cellular energy load [3] . Amino acids are the most potent activators of TOR in animals [21] , [22] . However, the established transducers of amino acid sensing to TOR in yeast and humans (the TOR-interacting proteins: RAG GTPase, TSC1/2, and RHEB) are absent in plants [23] . This raises the fundamental question if and how amino acid sensing is achieved in photo-autotrophic organisms, which, in contrast to animals, are able to synthesize all proteinogenic amino acids due to assimilation of inorganic carbon (C), nitrogen (N), and sulfur (S). In this study, we addressed the relevance of TOR for sensing of the amino acid cysteine in Arabidopsis thaliana . We focused on cysteine, since it is the central metabolite that coordinates the flux of sulfur with fluxes of carbon and nitrogen in all chemo-autotrophic and photo-autotrophic organisms. Our results provide evidence that the availability of cysteine precursors, rather than cysteine itself, is sensed by plants. This unique mechanism allows plants to distinguish between limitations of carbon/nitrogen (C/N) vs. limitation of sulfur (S) for amino acid biosynthesis. Selective sensing of precursor limitations for cysteine synthesis is accomplished in the C/N branch by GCN2 or in the S branch by Glc-TOR signaling. The differential activation of both sensor kinases regulates meristematic activity, translation efficiency, inorganic sulfur uptake, and remobilization of nutrients by autophagy to coordinate growth with nutrient limitation. The data reveal a specific adaptation of the TOR system to the photo-autotrophic lifestyle of plants. Impact of sulfide or OAS supply on translation and growth Synthesis of the sulfur-containing amino acid cysteine by O -acetylserine-(thiol)lyase (OAS-TL) is the sole entry point of reduced sulfur in the form of sulfide into plant metabolism, thereby coordinating the flux of sulfur with the fluxes of carbon and nitrogen [24] . Provision of sulfide by sulfite reductase (SiR) and the C/N precursor O -acetylserine (OAS) by serine acetyltransferase (SERAT) are known to limit cysteine synthesis in plants [25] , [26] , [27] , [28] (Fig. 1a ). In order to understand sensing of cysteine limitation in autotrophic eukaryotes, we used Arabidopsis thaliana to engineer a triple knockout plant ( serat tko ) that lacked the major SERAT isoforms in the cytosol (SERAT1;1), the plastids (SERAT2;1), and the mitochondria (SERAT2;2) and compared it to the sir1-1 knock-down plant (Fig. 1b and Supplementary Fig. 1a ). SERAT activity was unaffected in sir1-1 and decreased to 5 ± 2% (mean ± s.e.m.) of wild-type level in serat tko (Supplementary Fig. 1b ). The sir1-1 mutation decreased SiR abundance to 8 ± 4% (mean ± s.e.m.) of wild-type level. The SiR abundance was enhanced in serat tko strongly suggesting that sulfide supply by SiR is not co-downregulated in this mutant (Supplementary Fig. 1c ). Both mutants were impaired in cysteine synthesis and retarded in growth compared to wild type (Fig. 1b and Supplementary Fig. 1d ). Significantly lowered translation of proteins as determined by incorporation of glutamic acid into the total protein fraction in fully differentiated leaf cells was observed (Fig. 1c ). Fig. 1 Limitation of OAS or sulfide for Cys biosynthesis results in decreased translation and distinct metabolic phenotype. a Metabolic pathway of cysteine biosynthesis. b Rosette phenotype of 7-week-old wild-type serat tko and sir1-1 grown in hydroponic culture. Scale bar, 2 cm. c Global translation rate in different genotypes as determined by time-resolved incorporation of 3 H-glutamic acid into proteins ( n = 3, mean ± s.e.m., one-way ANOVA, * p < 0.05). d Relative fold change of metabolites is depicted as a heat map in cysteine-synthesis-depleted mutants compared to wild type ( n = 3–4, one-way ANOVA, * p < 0.05, ** p < 0.01) Full size image Limitation of sulfide or OAS triggers specific responses Next, we measured metabolite levels in the respective mutants to study the metabolic consequences of impaired SERAT or SiR activity (Fig. 1d ). Although both mutants suffered from impaired cysteine synthesis, they showed very different adaptions of primary metabolism due to limitation of either C/N precursor in serat tko mutants or sulfide in sir1-1 mutants. These specific adaptations occurred in photo-autotrophic (leaves) and heterotrophic tissue (roots) of both mutants, albeit to a different extent for individual compounds (Fig. 1d and Supplementary Fig. 1e ). In sir1-1 , the levels of several carbohydrates were downregulated, which in turn caused depletion of intermediates of the tricarboxylic acid (TCA) cycle in roots and leaves. Depletion of TCA cycle intermediates was not evident in serat tko and was corroborated by only marginally affected monosaccharide levels. Accordingly, the energy charge was specifically only lowered in shoots and roots of sir1-1 plants (Supplementary Fig. 1f ). These results indicate that carbon fixation into glucose and use of glucose in the TCA cycle was not downregulated due to decreased cysteine biosynthesis, but specifically in response to lowered sulfur assimilation in sir1-1 . OAS, the product of SERAT, and sulfate were decreased in leaves and roots of serat tko but accumulated in sir1-1 in accordance with the known regulatory link between OAS and the high-affinity uptake system for sulfate [24] . Cysteine steady state levels were only depleted in heterotrophic roots but kept constant in leaves of both mutants. The unexpected finding of unchanged cysteine pools in leaves ruled out the possibility that decreased translation in both mutants is a simple consequence of lowered cysteine pool size. Obviously, both mutants specifically sensed decreased cysteine precursor supply and responded in both cases with decreased growth and decreased translation in order to maintain the cysteine steady state level in leaves. Limitation of sulfide but not OAS decreases ribosomal RNA To uncover the specific signaling mechanisms in response to C/N precursor limitation or S-precursor limitation for cysteine in both mutants, we performed microarray-based expression profiling. The analysis of global transcriptome changes in roots of sir1-1 and serat tko revealed a specific response to OAS limitation for cysteine biosynthesis in serat tko and limited sulfur supply in sir1-1 (Fig. 2a ). An enrichment analysis of functional categories of the significantly regulated genes in sir1-1 (Fig. 2b, c and Supplementary Tables 1 and 2 ) and serat tko (Fig. 2d, e and Supplementary Tables 1 and 2 ) uncovered several commonly downregulated pathways, including protein processing in the ER and branched-chain amino acid degradation. Downregulation of these pathways is in agreement with the observed decreased translation rate in both mutants (Fig. 1c ). Specifically in sir1-1 , sulfur metabolism was significantly upregulated (Fig. 2b ). This included induction of the high-affinity sulfate transporters SULTR1;1 and SULTR1;2 and explained the strong accumulation of sulfate in sir1-1 (Fig. 1d ). The entire sulfur deficiency response (induction of sulfate uptake and sulfate reduction) was evidently absent in roots of serat tko (Supplementary Fig. 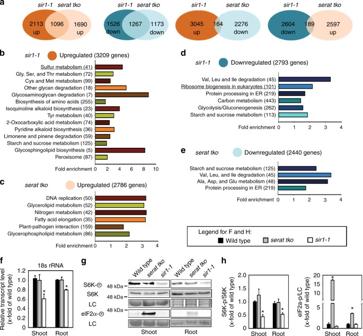Fig. 2 Specific sensing of C/N- or S-precursors for Cys results in distinct transcriptome reprogramming and specific translation regulation.aVenn diagrams andb–efunctional category analysis (p< 0.05, FDR < 0.25) for transcriptional response in roots of 7-week-oldserat tkoandsir1-1plants. The compared sets of genes contained transcripts, which were significantly (p< 0.05) up- or downregulated by more than 1.25-fold insir1-1orserat tkoin comparison to the wild type. The details of the highlighted categories with underlines are further presented in Supplementary Figs.2and4.fSpecific downregulation of 18s rRNA in response to sulfide limitation (n= 3, mean ± s.e.m., one-way ANOVA, *p< 0.05).gTOR and GCN2 activity was determined by antibodies against S6K-p, S6K (apparent sizes: 52 kDa) and eIF2α-p (apparent size: 43 kDa) andhcalculated by the ratio of S6K-p/S6K and eIF2α-p/LC in x-fold of wild type (n= 3, mean ± s.e.m., one-way ANOVA, *p< 0.05) 2 and Supplementary Table 2 ), which provides a functional explanation for the many differences observed in the metabolite fingerprints of both mutants (Fig. 1d and Supplementary Fig. 1e ). Fig. 2 Specific sensing of C/N- or S-precursors for Cys results in distinct transcriptome reprogramming and specific translation regulation. a Venn diagrams and b – e functional category analysis ( p < 0.05, FDR < 0.25) for transcriptional response in roots of 7-week-old serat tko and sir1-1 plants. The compared sets of genes contained transcripts, which were significantly ( p < 0.05) up- or downregulated by more than 1.25-fold in sir1-1 or serat tko in comparison to the wild type. The details of the highlighted categories with underlines are further presented in Supplementary Figs. 2 and 4 . f Specific downregulation of 18s rRNA in response to sulfide limitation ( n = 3, mean ± s.e.m., one-way ANOVA, * p < 0.05). g TOR and GCN2 activity was determined by antibodies against S6K-p, S6K (apparent sizes: 52 kDa) and eIF2α-p (apparent size: 43 kDa) and h calculated by the ratio of S6K-p/S6K and eIF2α-p/LC in x-fold of wild type ( n = 3, mean ± s.e.m., one-way ANOVA, * p < 0.05) Full size image In roots of sir1-1 , messenger RNAs (mRNAs) encoding for ribosome proteins and proteins associated with ribosome biogenesis accumulated to lower levels when compared to the wild type (Fig. 2c and Supplementary Fig. 3 ). The significant enrichment for downregulated transcripts related to ribosome biogenesis provides the most likely explanation for the decreased translation rate observed in sir1-1 (Fig. 1c ). Surprisingly, ribosome biogenesis was not affected in serat tko , although serat tko showed a similar phenotype to sir1-1 with respect to slower growth and decreased translation (Fig. 1b, c ). TOR regulates translation in sir1-1 but not in serat tko The specific downregulation of transcripts related to ribosome biogenesis prompted us to test the abundance of the 18S and 25S rRNAs. Only in sir1-1 , the abundances of these rRNAs were significantly decreased in shoots (18s rRNA: 61 ± 10%, 25s rRNA: 60 ± 2%, mean ± s.e.m.) and roots (18s rRNA: 79 ± 2%, 25s rRNA: 53 ± 7%, mean ± s.e.m., Fig. 2f and Supplementary Fig. 4 ). In plants, transcription of rRNAs and translation are under positive control of TOR [10] , [15] , which specifically phosphorylates the downstream kinase S6K at Thr 449 [3] , [29] . This phosphorylation is the canonical trigger for activation of ribosome biogenesis and translation in eukaryotes [3] . When we assayed the phosphorylation of S6K with a phospho-specific antiserum, we found it to be decreased by 56 ± 7% in shoots and 47 ± 6% in roots of sir1-1 . In contrast, serat tko displayed wild-type-like S6K phosphorylation levels (Fig. 2g, h ). In order to show the specificity of TOR downregulation by decreased SIR abundance, we tested two additional SiR mutants, KD1T ( sir1-3 ) and KD3P ( sir1-4 ) described in Yarmolinsky et al. [30] . The sir1-3 mutant was retarded in growth due to significantly lowered SiR abundance, whereas sir1-4 displayed wild-type-like phenotype and SiR protein level (Supplementary Fig. 5a–d ). In line with the observed SIR abundance in both lines, TOR activity was only decreased in sir1-3 but not in sir1-4 (Supplementary Fig. 5d, e ). These results suggest that significant downregulation of SiR in sir1-1 and sir1-3 causes downregulation of TOR activity as determined by phosphorylation of its downstream target S6K. Since serat tko plants have reduced translation rates (Fig. 1c ) but neither reduced 18S rRNA levels (Fig. 2f ) nor reduced TOR activity (Fig. 2h ), we tested if the reduced global translation in serat tko is caused by phosphorylation of the eukaryotic initiation factor eIF2α. Immunological detection of eIF2α phosphorylation revealed 17 ± 1 (mean ± s.e.m.) fold more abundance of the phosphorylated eIF2α protein in leaves and 3.6 ± 0.1 (mean ± s.e.m.) fold more in roots of serat tko when compared to wild type. Phosphorylation of eIF2α was not affected in sir1-1 (Fig. 2g, h ). In sum, sir1-1 mutants and serat tko appear to reduce global translation rates via two independent sensing mechanisms: in sir1-1 via downregulation of TOR, whereas in serat tko via elevated eIF2α phosphorylation. Sulfur deficiency decreases TOR activity and glucose levels In search for the molecular signal that triggers TOR inhibition after decreased S-precursor supply for cysteine biosynthesis in sir1-1 , we characterized the impact of sulfate deprivation on TOR and GCN2 activity. Sulfate deficiency caused specific decrease of TOR activity in leaves of wild-type plants, whereas the stress-related sensor–kinase GCN2 was not affected (Fig. 3a and Supplementary Fig. 6a ). In agreement with GCN2 not playing an important role in sulfate sensing, a GCN2 loss-of-function mutant was not more sensitive to sulfate deprivation and showed the same response as the wild type with respect to sulfur deficiency-induced metabolite adaptations (Supplementary Fig. 6b ). Fig. 3 Sulfur availability downregulates TOR activity and sugar metabolism. a Immunological detection of S6K-p, S6K (52 kDa) and eIF2α-p (43 kDa) with specific antisera was used for calculation of relative TOR activity by the ratio of S6K-p/S6K in x-fold of wild type ( n = 3, mean ± s.e.m., t -test, * p < 0.05). b 18s and 25s rRNA level were measured in the shoot of wild type under sulfur deficiency ( n = 3, mean ± s.e.m., t -test, * p < 0.05). c Growth phenotype of the des1-1 mutant having low sulfide level in the cytosol. Scale bar, 2 cm. d Immunological detection of S6K phosphorylation status in the genotypes shown in c (apparent sizes of S6K-p, S6K: 52 kDa). e Calculation of TOR activity by the ratio of S6K-p/S6K in x-fold of wild type ( n = 3, mean ± s.e.m., one-way ANOVA, * p < 0.05). f , g Functional category analysis ( p < 0.05, FDR < 0.25) for downregulated genes in shoots of 7-week-old sir1-1 and sulfur-deficient WT plants. The compared sets of genes contained transcripts, which were identified by microarray analysis to be significantly ( p < 0.05) downregulated by more than 1.25-fold. The categories related to sugar metabolism are highlighted with underlines. h Soluble sugar levels in shoots of 7-week-old sulfur-deficient plants ( n = 4, mean ± s.e.m., t -test, * p < 0.05) Full size image Inhibition of TOR by sulfate deprivation resulted in significantly lower amounts of 18S and 25S rRNA in the wild type (Fig. 3b ). Impairment of sulfur reduction by sulfate deprivation in the wild type or by the sir1-1 mutation could inhibit TOR by directly affecting the cytosolic sulfide concentration or by an unknown messenger. To test the first hypothesis, we determined TOR activity in the des1-1 mutant, which has previously been shown to possess low sulfide levels in the cytosol [31] . In our growth conditions, des1-1 grew like wild type and displayed TOR activity similar to wild type (Fig. 3c ). In contrast, sir1-1 produced less biomass, which is consistent with the lowered TOR activity in comparison to wild type and des1-1 (Fig. 3d, e ), making cytosolic sulfide levels an unlikely signal. In search for a potential messenger system that transmits the sulfide limitation signal from the chloroplasts to the cytosolic TOR sensor–kinase complex, we compared the transcriptional response of wild-type plants to sulfate deprivation with the transcriptional response of SiR-activity-depleted plants ( sir1-1 , Fig. 3f , g). We found that photosynthesis and several carbon metabolic routes are affected in the same way under both conditions (Fig. 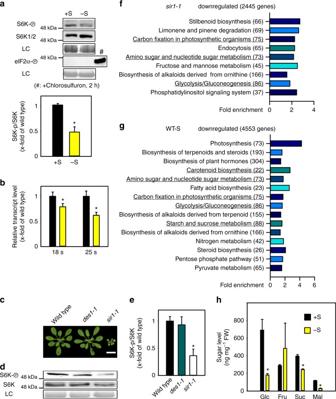Fig. 3 Sulfur availability downregulates TOR activity and sugar metabolism.aImmunological detection of S6K-p, S6K (52 kDa) and eIF2α-p (43 kDa) with specific antisera was used for calculation of relative TOR activity by the ratio of S6K-p/S6K in x-fold of wild type (n= 3, mean ± s.e.m.,t-test, *p< 0.05).b18s and 25s rRNA level were measured in the shoot of wild type under sulfur deficiency (n= 3, mean ± s.e.m.,t-test, *p< 0.05).cGrowth phenotype of thedes1-1mutant having low sulfide level in the cytosol. Scale bar, 2 cm.dImmunological detection of S6K phosphorylation status in the genotypes shown inc(apparent sizes of S6K-p, S6K: 52 kDa).eCalculation of TOR activity by the ratio of S6K-p/S6K in x-fold of wild type (n= 3, mean ± s.e.m., one-way ANOVA, *p< 0.05).f,gFunctional category analysis (p< 0.05, FDR < 0.25) for downregulated genes in shoots of 7-week-oldsir1-1and sulfur-deficient WT plants. The compared sets of genes contained transcripts, which were identified by microarray analysis to be significantly (p< 0.05) downregulated by more than 1.25-fold. The categories related to sugar metabolism are highlighted with underlines.hSoluble sugar levels in shoots of 7-week-old sulfur-deficient plants (n= 4, mean ± s.e.m.,t-test, *p< 0.05) 3f, g and Supplementary Table 3 ). Furthermore, carbon metabolism and glycolysis was specifically downregulated in roots of sir1-1 but not in roots of serat tko (Fig. 2c, e ). In plants, carbohydrates are mainly produced in chloroplasts by de novo fixation of CO 2 via photosynthesis but transported into the cytosol for further metabolization. Since glucose (Glc) and its metabolization in the TCA cycle is a well-established trigger of TOR in plants [11] , we determined the most abundant carbohydrates in leaves of sulfate-deprived wild-type plants. Specifically Glc, maltose (Glc-Glc), and sucrose (Glc-Fru) were downregulated, while fructose (Fru) was unaffected (Fig. 3h ). Also sir1-1 displayed a significant decrease of Glc and TCA cycle intermediates. Remarkably, Glc levels and TCA cycle intermediates were almost unaffected in serat tko (Fig. 1d ). Since limitation of sulfide supply by sulfate deprivation of the wild type or decreased SiR activity in sir1-1 resulted in decrease of soluble sugars and TOR activity, we analyzed TOR activity and sugar levels after short-term sulfide fumigation. Fumigation of sulfide for 6 h caused a strong increase of soluble sugars (Glc, Fru, Suc, and Mal) and TOR kinase activity (Supplementary Fig. 7 ), strongly indicating a positive correlation between sulfide level and soluble sugar level and TOR activity. Taken together, these results raise the possibility that reduced glucose metabolization provide the specific trigger for downregulation of TOR in sir1-1 and sulfur-deprived wild-type plants via the established glucose-TOR signaling [11] . Low glucose levels trigger inhibition of TOR in sir1-1 Roots and shoots of higher plants can independently produce sulfide and cysteine. In contrast, de novo fixation of carbon into carbohydrates is restricted to the shoot of plants. Grafting of sir1-1 shoots to wild-type roots induced a sir1-1 -like growth phenotype in wild-type roots, although these roots have the capacity to produce sulfide. Vice versa, grafting of wild-type shoots to sir1-1 roots complemented the sir1-1 root phenotype (Fig. 4a and Supplementary Fig. 8 ). These results further strengthen the hypothesis that downregulation of carbohydrate production in sir1-1 shoots is the signal for TOR inhibition and that it controls TOR activity in sir1-1 roots via phloem-mediated transport of sucrose as it has been suggested earlier for photosynthesis-induced TOR activation in roots [11] . Since grafting of sir1-1 roots to wild-type shoots did not cause decreased growth of leaves, a potential root-to-shoot signal generated by low cysteine levels in roots of sir1-1 is unlikely. Fig. 4 Sulfur availability regulates root meristem and plant growth via glucose-TOR. a Phenotype of chimeric plants obtained by grafting of wild-type (WT) and sir1-1 organs. Identity of organs is depicted as shoot/root. Scale bar, 2 cm. b – e Feeding of serat tko and sir1-1 seedlings with glucose. b Immunological detection of S6K-p, S6K (apparent sizes: 52 kDa), and eIF2α-p (apparent size: 43 kDa) with specific antisera in wild-type serat tko and sir1-1 . c , d Phenotype of wild-type serat tko and sir1-1 plants in the absence and presence of glucose. Scale bar, 1 cm. e Impact of glucose on root meristem activity in wild-type serat tko and sir1-1 . Scale bar, 25 µm. f Root meristem activity of 7-day-old WT seedlings treated with TOR inhibitor (AZD-8055) or GCN2 activator (Chlorosulfuron, CHL) for 2 h. Scale bar, 25 µm Full size image In order to provide direct functional evidence for the regulation of TOR by Glc in sir1-1 , we fed Glc to both cysteine-synthesis-depleted mutants. As expected, Glc application increased TOR activity in sir1-1 significantly (Fig. 4b and Supplementary Fig. 9a ). The enhanced TOR activity restored growth of shoot and of root and resulted in an almost wild-type-like phenotype of the Glc/Suc-treated sir1-1 seedling (Fig. 4c, d and Supplementary Fig. 9b ). The dwarf growth of sir1-3 was also rescued by exogenous glucose feeding (Supplementary Fig. 9c, d ). In contrast, the growth of serat tko was not affected by Glc application, since Glc did not affect eIF2α-phosphorylation (Fig. 4b ). TOR is an important regulator of stem cell activation in plants [32] . Consequently, meristematic activity of sir1-1 roots was found to be significantly lower when compared with wild type and serat tko , due to inhibition of TOR in sir1-1 . Application of Glc or sucrose—the phloem-mobile shoot-to-root carrier of Glc—restored meristematic activity and thus provides a molecular explanation for the significant growth stimulation of Glc-treated sir1-1 seedlings (Fig. 4e and Supplementary Fig. 10a, b ) that restored 87 ± 4% (mean ± s.e.m.) of biomass production by the wild type (Supplementary Fig. 8d ). Glc-induced root meristem reactivation in sir1-1 was prevented by short-term inhibition of mitochondrial respiration or TOR activity (Supplementary Fig. 10c ). In contrast, upregulation of eIF2α-phosphorylation in serat tko had no impact on meristematic activity (Fig. 4e ). Also activation of GCN2 by chlorsulfuron application [8] did not affect root meristem activity (Fig. 4f and Supplementary Fig. 10d ). In search for a TOR-independent functional explanation of the retarded growth phenotype of serat tko , we determined the cell size of wild-type serat tko and sir1-1 and identified diminished cell elongation as a significant contributor to the smaller serat tko appearance (Supplementary Fig. 11 ). Limited S supply for Cys synthesis induces autophagy TOR is a well-established negative regulator of autophagy in metazoa, but its function in plants is less characterized [33] . Therefore, we treated Arabidopsis roots with the highly specific TOR inhibitor AZD-8055. Application of AZD-8055 caused a fast drop in phosphorylation of S6K and induced autophagy within 2 h, as demonstrated by lipidation of the autophagosome marker ATG8a (Supplementary Fig. 12a ). The ribosomal RNA was decreased to 21 ± 3% of control level after 6 h of TOR inhibition (Supplementary Fig. 12b ). The phosphorylation of eIF2α was unaffected for up to 6 h of AZD-8055 treatment (Supplementary Fig. 12a ), which is in agreement with unchanged GCN2 activity in TOR overexpression and TOR-RNAi lines [8] . Since TOR is significantly downregulated in sir1-1 , we tested if autophagy is also induced in this mutant. Lipidation of ATG8a (Fig. 5a, b ), degradation of the selective autophagy cargo receptor neighbor of BRCA1 (NBR1, Fig. 5a , b) and fluorescent staining of acidic autophagosomes (Fig. 5c ) demonstrated a significant upregulation of autophagy in sir1-1 leaves and roots. Autophagy was not induced in serat tko plants. From these findings, we presumed that decrease of TOR activity by impairment of sulfate reduction might also trigger autophagy induction under sulfate deprivation. Indeed, sulfate deficiency significantly induced autophagy in leaves of wild-type plants as shown by ATG8 lipidation (Fig. 5d ). Taken together, these results uncover the importance of enhanced autophagy for remobilization of internal resources during sulfur deprivation and that the trigger for induction of autophagy under sulfur deprivation is the decreased TOR activity due to lowered S-precursor supply for cysteine biosynthesis. Fig. 5 Autophagy is specifically induced by limited S-precursor supply for cysteine biosynthesis. a Autophagy induction in the shoot of serat tko and sir1-1 was determined by immunological detection of the canonical autophagy marker ATG8a and NBR1 with specific antisera. Lipidation of ATG8a (ATG8a-PE) (apparent size: 15–20 kDa) is essential for autophagosome formation and indicated by a significant shift during electrophoresis. NBR1 is a cargo receptor for selective autophagy and consequently degraded in autophagic bodies (D-NBR1) (apparent size: 50–75 kDa). b Level of ATG8a-PE and D-NBR1 shown in a were quantified ( n = 3, mean ± s.e.m., one-way ANOVA, * p < 0.05). c Autophagy induction in the root of serat tko and sir1-1 was detected by MDC staining. White arrows marked the visible autophagic bodies. Scale bar, 25 µm. d Autophagy induction in the shoot of WT under sulfur deficiency was determined by ATG8a-PE level ( n = 3, mean ± s.e.m., t -test, * p < 0.05) Full size image Eukaryotic cells invest significant resources in protein translation and have therefore established sophisticated mechanisms to regulate this process in response to growth stimuli and nutrient supply. In the heart of this regulation lies the sensor–kinase TOR. The most comprehensive signaling network of TOR is found in humans. It consists of two sensory protein complexes mTORC1 and mTORC2, which perceive signals from growth factors and diverse nutrient stimuli [34] . Direct sensing of amino acid levels via the Rag-TSC2-Rheb axis is one of the most important functions of TOR in humans [35] . This mechanism is largely conserved in fungi and orthologous proteins of this axis are present in opisthokonts [22] , [36] , [37] . In contrast, we show here that plants do not directly sense the concentration of the amino acid cysteine but the supply of its precursors. In plants as photo-autotrophic organisms, cysteine is the metabolic hub that integrates the products of reductive assimilation of sulfate, nitrate, and CO 2 . The reason for the conceptually different approach of TOR function apparently is to allow plants to distinguish which building blocks from the S or the C/N assimilation pathways for cysteine synthesis are limiting and to respond in a highly specific manner to changing demands. The absence of a direct cysteine-sensing mechanism is consistent with the previously observed lack of TOR activation after application of an amino acid cocktail including cysteine [11] . It is remarkable in this context that the last common eukaryotic ancestor evidently possessed orthologs for RAG, TSC2, and Rheb [36] , strongly indicating a specific loss of this signaling mechanism in the plant lineage of eukaryotes. Further plant-specific adaptions of the TOR signaling network are indicated by the absence of mTORC2 components in plants [36] . In search for the direct-sensing mechanism of the cysteine precursors, we identified GCN2 as the sensor for the supply via the C/N branch. This finding was unexpected due to the general role of GCN2 as an amino acid sensor in eukaryotes and the conserved mechanism from human to plants for activation of GCN2 by uncharged tRNAs [6] , [9] , [38] . However, GCN2 was not responding to sulfur limitation and decrease of cysteine levels in sir1-1 roots, but was specifically activated by limitation of C/N supply for cysteine production by a so far unknown mechanism. Consequently, GCN2 did not contribute to regulation of the sulfur deficiency response. The downregulation of TOR activity in the sir1-1 mutant and during sulfur deficiency in the wild type demonstrated that the sensing of the precursor supply of the S branch takes place via this sensor–kinase. In search for the signal that links S-precursor supply with TOR activity, we observed that glucose feeding ameliorated the S-deficiency phenotype of sir1-1 and that decreased flux through the sulfate assimilation pathway in sir1-1 or sulfate-deprived wild type resulted in downregulation of glucose bioenergetics. Furthermore, short-term sulfide fumigation caused fast and significant upregulation of glucose levels and TOR activity. Indeed, regulation of plant TOR by glucose was previously reported and requires glucose metabolization by the TCA cycle [11] . This finding explains the failure of glucose to trigger meristem reactivation in sir1-1 when mitochondrial respiration or TOR inhibitors were co-applied with glucose. In humans, low energy/glucose levels inhibit mTORC1 by activation of the AMP-activated kinase (AMPK), which in turn phosphorylates RAPTOR (regulatory-associated protein of TOR) [39] . The plant AMPK homolog, SnRK1.1, is not responding to high AMP levels but is activated by low levels of trehalose-6-phosphate (Tre6P). Tre6P is synthesized from glucose and acts as a general carbon status signal in plants, since its concentration tightly follows glucose metabolization [40] . SnRK1.1 phosphorylates plant RAPTOR1B and its overexpression caused decreased phosphorylation of TOR substrates [41] . Consequently, the observed sulfur deficiency-induced low-glucose levels might have been sensed by SnRK1 that inhibited plant mTORC1 activity by phosphorylation of RAPTOR1B. Furthermore, short-term sulfide fumigation increases glucose levels and TOR activity, which is in agreement with the proposed role of the glucose-TOR signaling under sulfur deprivation. However, these data do not exclude a direct regulation of TOR by sulfide via a so far unknown mechanism. The TOR-mediated response to sulfur deficiency included induction of autophagy for remobilization of internal resources, lowered translation, and inhibition of meristem activity. Many of these reactions have also been shown to occur upon deprivation of other nutrients, possibly suggesting a general role of TOR in nutrient sensing of plants. In particular, the control of meristem activity by nutrient availability is crucial, since developmental plasticity of the root system is a hallmark of many mineral nutrient-deficiency responses [42] . In line with the idea that TOR is a central regulator of meristem activity and consequently developmental plasticity in response to environmental cues, TOR has been evidenced recently to participate in the light-induced activation of the shoot apical meristem [32] . The surprising finding of differential activation of TOR and GCN2 by supply of distinct cysteine precursors provides the molecular framework for specific responses of plants toward diverse nutrient limitations and adds novel mechanistic insights into the homeostatic regulation of the macronutrient sulfur. We anticipate that the here-uncovered knowledge will stimulate research on regulation of other mineral nutrients and have profound impact on future breeding strategies to enhance nutrient use efficiency of crop plants, one of the currently most important traits of commercial breeding programs. Plant genotypes and growth conditions Arabidopsis thaliana mutant plants, as well as wild-type control plants were in the Columbia (Col-0) ecotype. Wild-type plants (N1092) and salk_103855 ( des1-1 ) were gained from the Nottingham Arabidopsis Stock Centre. The triple-mutant serat1;1 serat2;1 and serat2;2 ( serat tko ) was constructed by crossing single serat T-DNA knock-out lines. The T-DNA insertion line sir1-1 was described previously [25] . sir1-3 (salk_075776, KD1T [30] ) and sir1-4 (sail_1223C03, KD3P [30] ) were gained from Prof. Moshe Sagi (Weizmann Institute of Science, Israel). The gcn2 mutant (GABI_862B02) was provided by Prof. Jean-Marc Deragon (University of Perpignan, France). If not otherwise indicated, plants were grown under short-day conditions for 2 weeks [25] . Then seedlings were transferred into larger pots containing 15 L half-strength Hoagland solution (pH 5.8) either supplemented with 500 µM MgSO 4 (normal sulfate condition) or 1 µM MgSO 4 (-S) for 5 weeks and were transferred to fresh media 24 h before being harvested. Glucose-feeding experiment was performed with seedlings grown on AT medium (pH 5.8, 0.6% agar) supplemented with 30 mM Glc. All plants were grown in a short-day climate chamber (8.5 h light/15.5 h dark; 80–100 μmol m −2 s −1 ; 22 °C day/18 °C night; 50% humidity). Chemical inhibitor treatment was performed with media containing AZD-8055 (5 µM) or chlorosulfuron (0.5 µM) for 2 h. Determination of translation Leaf discs were incubated for 30, 60, and 90 min with radiolabeled 3H-glutamic acid (10 μCi ml −1 ). After incubation, proteins were extracted and desalted using PD SpinTrap G-25 columns (GE Healthcare Life Science) to remove the non-incorporated 3 H-glutamic acid. To quantify incorporated radiolabeled glutamic acid into proteins, leaflets were dissolved in 10 ml scintillation liquid (Ultima Gold; Perkin Elmer) and counted for 5 min with the liquid scintillation analyzer Tri-Carb 2810TR (PerkinElmer). Determination of metabolites Soluble sugars were extracted by 80% ethanol and separated on Dionex ICS-3000 system with CarboPac PA1 with CarboPac PA1-Guard column at 25 °C. For the measurement of amino acids, thiols, and OAS, total metabolites were extracted from 50 mg leaf or root materials with 500 µl 0.1 M HCl. Determination of amino acids and OAS was based on the derivatization with the fluorescent dye AccQ-TagTM. An aliquot of 10 µl HCL extracts was mixed with 70 µl borate buffer (0.2 M, pH 8.8) and 20 µl 3 mg ml −1 AccQ-TagTM solution. The derivatization was performed at 55 °C for 10 min. The separation of amino acids was performed by reversed phase HPLC on a Nova-PakTM C18, 3.9 × 150 mm column. Derivatives were detected at an emission wavelength of 395 nm upon excitation at 250 nm. The data were analyzed using the software Empower Pro. To detect thiols, 25 μl HCl extracts were incubated with 245 μl reduction buffer (68 mM Tris, pH 8.3; 0.34 mM DTT; 25 μl 0.08 M NaOH) for 1 h at room temperature in the dark. Free thiol groups were released and derivatized with 0.85 mM MBB at room temperature for 15 min in the dark. An aliquot of 705 µl 5% acetic acid was used to stop the derivatization. The separation of thiols was performed by reversed phase HPLC on a Nova-PakTM C18, 4.6 × 250 mm column. Thiol-bimane derivatives were detected at an emission wavelength of 480 nm upon excitation at 380 nm. Ions were extracted from 50 mg materials in 300 µl ddH 2 O. The extraction was carried out at 98 °C for 30 min under constant shaking. The aqueous extracts were diluted three times with ddH 2 O to a final volume of 300 µl and transferred to HPLC vials (Dionex). The determination was carried out on a system ICS-3000 (Dionex) with an IonPac AS 11 column and 15–300 mM NaOH (Fluka, in ddH2O) as eluent. Quantitative calculation of the organic acids and ions was performed using Chromeleon software 6.7 (Dionex). Immunological detection of proteins For immunological detection of S6K-p and eIF2α-p, total soluble proteins were extracted from 50 mg plant materials with 250 µl 2× Laemmli buffer supplemented with 1% phosphatase inhibitor cocktail 2 (Sigma). Proteins were denatured for 5 min at 95 °C and separated on 10% SDS-PAGE. For immunological detection of S6K1/2, ATG8a-PE and NBR1, total proteins were extracted from 50 mg plant materials with 100 µl urea buffer (4 M urea, 100 mM DTT and 1% Triton X-100). Proteins were separated on 15% SDS-PAGE supplemented with 8 M urea. Subsequently, proteins were blotted to nitrocellulose membrane. The primary antibodies anti-S6k-p (Phospho-p70 S6 Kinase (p-Thr389), Cell Signaling, #9205, 1:5000), anti-S6K1/2 (Agrisera, #AS12-1855, 1:5000), eIF-2α Phospho (Epitomics, #1090-1, 1:10,000), anti-ATG8a-PE (Agrisera, #AS14-2811, 1:2000), and anti-NBR1 (Agrisera, #AS14-2805, 1:5000) were detected using the HRP-conjugated secondary antibody (1:30,000). The band intensity was quantified by Image Quant LAS4000 version 1.21 and normalized by the loading control. Full scans of blots are presented in Supplementary Fig. 13 . Microarray analysis Gene expression profiling was performed using an A. thaliana genechip (Aragene-1_0-st-typ) from Affymetrix (High Wycombe, UK). RNA was isolated from 100 mg homogenized leaf or root material of 7-week-old hydroponically grown plants with the peqGold total RNA Kit (Peqlab) according to the manufacturer’s protocol. DNA digestion was performed with the peqGOLD DNase I Digest Kit (Peqlab). All further steps were conducted by the collaboration partner Core-Lab for microarray analysis (Centre for medical research (ZMF); University of Mannheim): Biotinylated antisense cRNA was prepared according to the Affymetrix standard labeling protocol. Hybridization on the chip was conducted on a GeneChip Hybridization oven 640, subsequently dyed in the GeneChip Fluidics Station 450 and thereafter scanned with a GeneChip Scanner 3000. The entire equipment set was provided by the Affymetrix-Company (Affymetrix, High Wycombe, UK). Arrays were annotated using a custom CDF Version 17 with TAIR-IDs-based gene definitions. The raw fluorescence intensity values were normalized applying quantile normalization. Differential gene expression was analyzed based on log-linear mixed model ANOVA, using a commercial software package SAS JMP7 Genomics, version 6, from SAS (SAS Institute, Cary, NC, USA). A false-positive rate of a = 0.05 with FDR correction was taken as the level of significance. Functional category analysis by DAVID [43] was used to determine whether defined lists (or sets) of genes exhibit a statistically significant bias in their distribution within a ranked gene list (fold change cut: 1.25, p < 0.05, FDR < 0.25). 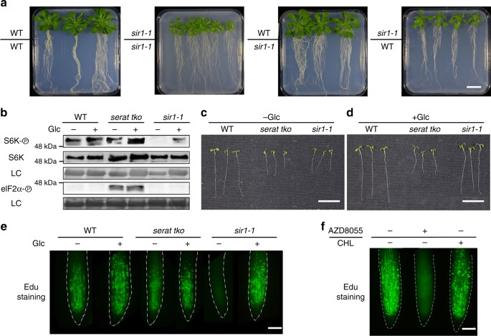Fig. 4 Sulfur availability regulates root meristem and plant growth via glucose-TOR.aPhenotype of chimeric plants obtained by grafting of wild-type (WT) andsir1-1organs. Identity of organs is depicted as shoot/root. Scale bar, 2 cm.b–eFeeding ofserat tkoandsir1-1seedlings with glucose.bImmunological detection of S6K-p, S6K (apparent sizes: 52 kDa), and eIF2α-p (apparent size: 43 kDa) with specific antisera in wild-typeserat tkoandsir1-1.c,dPhenotype of wild-typeserat tkoandsir1-1plants in the absence and presence of glucose. Scale bar, 1 cm.eImpact of glucose on root meristem activity in wild-typeserat tkoandsir1-1. Scale bar, 25 µm.fRoot meristem activity of 7-day-old WT seedlings treated with TOR inhibitor (AZD-8055) or GCN2 activator (Chlorosulfuron, CHL) for 2 h. Scale bar, 25 µm 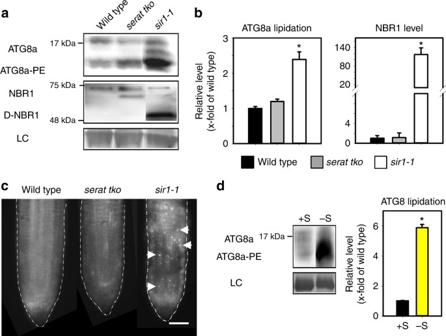Fig. 5 Autophagy is specifically induced by limited S-precursor supply for cysteine biosynthesis.aAutophagy induction in the shoot ofserat tkoandsir1-1was determined by immunological detection of the canonical autophagy marker ATG8a and NBR1 with specific antisera. Lipidation of ATG8a (ATG8a-PE) (apparent size: 15–20 kDa) is essential for autophagosome formation and indicated by a significant shift during electrophoresis. NBR1 is a cargo receptor for selective autophagy and consequently degraded in autophagic bodies (D-NBR1) (apparent size: 50–75 kDa).bLevel of ATG8a-PE and D-NBR1 shown inawere quantified (n= 3, mean ± s.e.m., one-way ANOVA, *p< 0.05).cAutophagy induction in the root ofserat tkoandsir1-1was detected by MDC staining. White arrows marked the visible autophagic bodies. Scale bar, 25 µm.dAutophagy induction in the shoot of WT under sulfur deficiency was determined by ATG8a-PE level (n= 3, mean ± s.e.m.,t-test, *p< 0.05) Determination of rRNA levels Levels of rRNAs were detected by qRT-PCR after cDNA conversion with specific primers 18s rRNA_RT and 25s rRNA_RT (Supplementary Table 4 ) by RevertAid H-Minus First Strand cDNA Synthesis Kit (Fermentas). qRT-PCR was performed with Rotor-Gene SYBR Green PCR Kit (Qiagen) and primers listed in Supplementary Table 4 (detailed method in Supplementary Methods). Determination of root meristem activity Edu (5-ethynyl-2′-deoxyuridine) staining was performed using Click-iT ® EdU AlexaFluor ® 488 Imaging Kit (Invitrogen). Seven-day-old seedlings grown on AT medium (pH 5.8, 0.6% agar) supplemented with 30 mM Glc were transferred to AT medium supplemented with 30 mM Glc and 5 µM AZD-8055 or 0.5 µM chlorsulfuron for 2 h. Then 5 µl 1 μM EdU in liquid AT medium was added directly on the root tip. The root tips were incubated with EdU for 30 min in the climate chamber. Then the seedlings were fixed in 100 μl fixation/permeabilization reagent (4% formaldehyde, 0.1% Triton X-100 in 1× PBS) for 30 min. After fixation, seedlings were incubated in the dark with 100 μl Click-iT reaction cocktail (prepared according to the manufacturer’s protocol, Click-iT ® EdU AlexaFluor ® 488 Imaging Kit, Invitrogen). The seedlings were washed with PBS buffer for two times. All the samples were analyzed by Leica DM IRB epifluorescent microscope with FITC/GFP filter (AlexaFluor 488: excitation 495 nm; emission 519 nm). Images were recorded by Leica DFC350 FX camera. Micro-grafting The grafting was performed with 7-day-old seedlings grown on ¼ MS media containing 1% sucrose, 1.4% agar, and 40 mg l −1 ampicillin. Shoot and root stocks were grafted and fixed together in a silicon tube (0.3 mm diameter, 3 mm length). Survived grafted plants were kept in the same growth condition for 5 weeks. MDC staining Seven-day-old seedlings were incubated with 50 µM MDC (Monodansylcadaverine, Sigma) in PBS buffer (137 mM NaCl, 2.7 mM KCl, 10 mM Na 2 HPO 4 , 1.8 mM KH 2 PO 4 ) for 15 min. Then the seedlings were washed with PBS buffer for two times and imaged by Leica DM IRB epifluorescent microscope with UV filter. Images were recorded by Leica DFC350 FX camera. Data availability Microarray data that support the findings of this study have been deposited in Gene Expression Omnibus database with the primary accession codes GSE93047, GSE93048, and GSE93049 ( http://www.ncbi.nlm.nih.gov/geo/GSE93047 ). The authors declare that all other data supporting the findings of this study are available within the paper and its supplementary information files.